Genotyping with CRISPR-Cas-derived RNA-guided endonucleases Restriction fragment length polymorphism (RFLP) analysis is one of the oldest, most convenient and least expensive methods of genotyping, but is limited by the availability of restriction endonuclease sites. Here we present a novel method of employing CRISPR/Cas-derived RNA-guided engineered nucleases (RGENs) in RFLP analysis. We prepare RGENs by complexing recombinant Cas9 protein derived from Streptococcus pyogenes with in vitro transcribed guide RNAs that are complementary to the DNA sequences of interest. Then, we genotype recurrent mutations found in cancer and small insertions or deletions (indels) induced in cultured cells and animals by RGENs and other engineered nucleases such as transcription activator-like effector nucleases (TALENs). Unlike T7 endonuclease I or Surveyor assays that are widely used for genotyping engineered nuclease-induced mutations, RGEN-mediated RFLP analysis can detect homozygous mutant clones that contain identical biallelic indel sequences and is not limited by sequence polymorphisms near the nuclease target sites. RGENs are derived from the adaptive immune system in bacteria and archaea known as clustered, regularly interspaced, short palindromic repeats (CRISPR)/CRISPR-associated protein (Cas) [1] ; they now belong to a family of genome-editing engineered nucleases that induce site-specific DNA cleavages in cells and organisms, whose repair via endogenous DNA double-strand break (DSB) repair systems gives rise to targeted mutagenesis [2] , [3] and chromosomal rearrangements [4] , [5] . Unlike zinc-finger nucleases (ZFNs) or transcription activator-like effector (TALE) nucleases (TALENs), whose DNA sequence specificities are determined by protein moieties, RGENs recognize and cleave DNA in a targeted manner using two separate components, that is, a small RNA component termed CRISPR RNA (crRNA) or single-chain guide RNA (sgRNA) that hybridizes with a 20-base pair (bp) long target DNA sequence and the Cas9 protein, derived from Streptococcus pyogenes , which recognizes the NGG (or, to a lesser extent, NAG [6] ) trinucleotide sequence known as the protospacer-adjacent motif (PAM). Thus, an RGEN site can be shown as 5′-X 20 NGG-3′, where X 20 corresponds to the crRNA sequence and N is any base. RGENs consist of Cas9, invariable transactivating crRNA (tracrRNA) and target-specific crRNA (or sgRNA that consists of essential portions of tracrRNA and crRNA), and are readily reprogrammed by replacing crRNA (or sgRNA) [7] . We and others have recently used RGENs for genome engineering in bacteria [8] , mammalian cells [9] , [10] , [11] , [12] , animals [13] , [14] , [15] , [16] , [17] , [18] , [19] and plants [20] , [21] , [22] . Engineered nuclease-induced mutations are detected by various methods, which include mismatch-sensitive Surveyor or T7 endonuclease I (T7E1) assays [23] , RFLP analysis [24] , fluorescent PCR [25] , DNA melting analysis [26] and Sanger and deep sequencing. The T7E1 and Surveyor assays are widely used but often underestimate mutation frequencies because the assays detect heteroduplexes (formed by the hybridization of mutant and wild-type sequences or two different mutant sequences); they fail to detect homoduplexes formed by the hybridization of two identical mutant sequences. Thus, these assays cannot distinguish homozygous bialleic mutant clones from wild-type cells nor heterozygous biallelic mutants from heterozygous monoalleic mutants ( Fig. 1a,b ). In addition, sequence polymorphisms near the nuclease target site can produce confounding results because the enzymes can cleave heteroduplexes formed by hybridization of these different wild-type alleles. RFLP analysis is free of these limitations and therefore is a method of choice. Indeed, RFLP analysis was one of the first methods used to detect engineered nuclease-mediated mutations [24] . Unfortunately, however, it is limited by the availability of appropriate restriction sites. 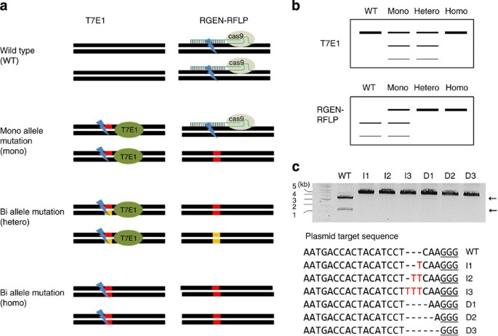Figure 1: Overview of RGEN-RFLP analysis. (a) A conceptual diagram of the T7E1 and RGEN-RFLP assays. Comparison of assay cleavage reactions in four possible scenarios after engineered nuclease treatment in a diploid cell: (WT) wild type, (Mono) a monoallelic mutation, (Hetero) different biallelic mutations and (Homo) identical biallelic mutations. Black lines represent PCR products derived from each allele; yellow and red boxes indicate insertion/deletion mutations generated by non-homologous end-joining. (b) Expected results of T7E1 and RGEN digestion resolved by electrophoresis. (c)In vitrocleavage assay of a linearized plasmid containing theC4BPBtarget site bearing indels. DNA sequences of individual plasmid substrates (bottom panel). The PAM sequence is underlined. Inserted bases are shown in red. Arrows (upper panel) indicate expected positions of DNA bands cleaved by the wild-type-specific RGEN after electrophoresis. Figure 1: Overview of RGEN-RFLP analysis. ( a ) A conceptual diagram of the T7E1 and RGEN-RFLP assays. Comparison of assay cleavage reactions in four possible scenarios after engineered nuclease treatment in a diploid cell: (WT) wild type, (Mono) a monoallelic mutation, (Hetero) different biallelic mutations and (Homo) identical biallelic mutations. Black lines represent PCR products derived from each allele; yellow and red boxes indicate insertion/deletion mutations generated by non-homologous end-joining. ( b ) Expected results of T7E1 and RGEN digestion resolved by electrophoresis. ( c ) In vitro cleavage assay of a linearized plasmid containing the C4BPB target site bearing indels. DNA sequences of individual plasmid substrates (bottom panel). The PAM sequence is underlined. Inserted bases are shown in red. Arrows (upper panel) indicate expected positions of DNA bands cleaved by the wild-type-specific RGEN after electrophoresis. Full size image Here we present a novel method of detecting and quantifying engineered nucleases-induced mutations in cultured cells and organisms by employing RGENs in RFLP analysis. Unlike T7E1 or Surveyor assays, RGEN-mediated RFLP analysis can distinguish homozygous bialleic mutant clones from wild-type cells and is not limited by sequence polymorphisms near the nuclease target sites. In addition, we show that RGEN-RFLP analysis can be used to genotype naturally-occurring indels and cancer-associated mutations in human cell lines. RGEN-mediated RFLP analysis We reasoned that RGENs can be employed in RFLP analysis, bypassing the use of conventional restriction enzymes. New RGENs with desired DNA specificities can be readily created by replacing crRNA; no de novo purification of custom proteins is required once recombinant Cas9 protein is available. Engineered nucleases, including RGENs, induce small insertions or deletions (indels) at target sites when the DSBs caused by the nucleases are repaired by error-prone non-homologous end-joining. RGENs that are designed to recognize the target sequences cleave wild-type sequences efficiently but cannot cleave mutant sequences with indels ( Fig. 1a,b ). We first tested whether RGENs can differentially cleave plasmids that contain wild type or modified C4BPB target sequences that harbour 1- to 3-base indels at the cleavage site. None of the six plasmids with these indels were cleaved by a C4BPB -specific RGEN [9] composed of target-specific crRNA, tracrRNA and recombinant Cas9 protein ( Fig. 1c ). In contrast, the plasmid with the intact target sequence was cleaved efficiently by this RGEN. Genotyping indels induced by RGENs via RGEN-RFLP analysis To test the feasibility of using RGEN-mediated RFLP (RGEN-RFLP in short) analysis for the detection of RGEN-induced mutations, we utilized K562 human cancer cell clones that had been modified at the C4BPB locus using the C4BPB -targeting RGEN. Among five C4BPB mutant clones we analysed, four clones had both wild-type and mutant alleles (heterozygous +/−) and one clone (#5) had only mutant alleles (compound heterozygous) ( Fig. 2a ). All of the mutations that occurred in these clones resulted in the loss of the RGEN target site. Thus, when the C4BPB mutant clones were subjected to RGEN genotyping, PCR amplicons of heterozygous +/− clones that contained both wild-type and mutant alleles were partially digested, and those of compound heterozygous −/− clones that did not contain the wild-type allele were not digested at all ( Fig. 2a ). In line with the plasmid digestion results, even a single-base insertion at the target site blocked the digestion of amplified mutant alleles by the C4BPB RGEN, showing the high specificity of RGEN genotyping. In contrast, the PCR products amplified from wild-type genomic DNA were digested completely by the RGEN. We subjected the PCR amplicons to the mismatch-sensitive T7E1 assay in parallel. Notably, the T7E1 assay failed to distinguish the compound heterozygous clone (#5) from the four +/− clones. 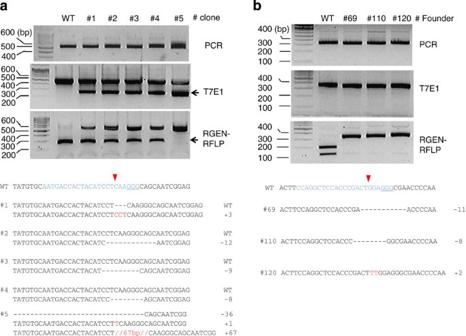Figure 2: Genotyping of RGEN-induced mutations via the RGEN-RFLP technique. (a) Analysis ofC4BPB-disrupted clones using RGEN-RFLP and T7E1 assays. Arrows indicate expected positions of DNA bands cleaved by RGEN or T7E1. The RGEN target site is shown in blue. Red arrows indicate the RGEN cleavage site. The PAM sequence is underlined. The number of inserted or deleted bases is shown. (b) Analysis of mouse founders that carried RGEN-induced homozygous biallelic mutations at theFoxn1gene using RGEN-RFLP and T7E1 assays. Figure 2: Genotyping of RGEN-induced mutations via the RGEN-RFLP technique. ( a ) Analysis of C4BPB -disrupted clones using RGEN-RFLP and T7E1 assays. Arrows indicate expected positions of DNA bands cleaved by RGEN or T7E1. The RGEN target site is shown in blue. Red arrows indicate the RGEN cleavage site. The PAM sequence is underlined. The number of inserted or deleted bases is shown. ( b ) Analysis of mouse founders that carried RGEN-induced homozygous biallelic mutations at the Foxn1 gene using RGEN-RFLP and T7E1 assays. Full size image We also used RGEN-RFLP to analyse three mutant mice that had been created by injecting a Foxn1 -targeting RGEN into one-cell stage embryos [19] . These founder mice carried identical biallelic mutations at the target site ( Fig. 2b ). As expected, the T7E1 assay failed to distinguish these homozygous mutant clones from the wild-type control, because annealing of the same mutant sequences forms homoduplexes. In contrast, the RGEN used for the creation of these mice successfully distinguished them from the wild-type control: The RGEN cleaved the PCR products amplified from wild-type genomic DNA completely but did not cleave those amplified from the mutants at all. Thus, RGEN-RFLP analysis has a critical advantage over the conventional mismatch-sensitive nuclease assay in the analysis of clones containing mutations induced by engineered nucleases. We also investigated whether RGEN-RFLP analysis is a quantitative method. Genomic DNA samples isolated from the C4BPB null clone and the wild-type cells were mixed at various ratios and used for PCR amplifications. The PCR products were subjected to RGEN genotyping and the T7E1 assay in parallel ( Fig. 3 ). As expected, DNA cleavage by the RGEN was proportional to the wild type to mutant ratio. In contrast, results of the T7E1 assay correlated poorly with mutation frequencies inferred from the ratios and were inaccurate, especially at high mutant %, a situation in which complementary mutant sequences can hybridize with each other to form homoduplexes. 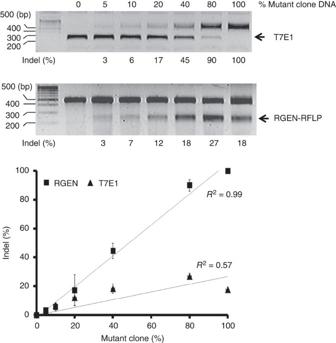Figure 3: Quantitative comparison of RGEN-RFLP analysis with T7E1 assays. Genomic DNA samples from wild type andC4BPB-disrupted K562 cells (clone #5 inFig. 2a) were mixed in various ratios and subjected to RGEN-RFLP and T7E1 assays. Data points are represented as mean±s.e.m. of two independent experiments. Figure 3: Quantitative comparison of RGEN-RFLP analysis with T7E1 assays. Genomic DNA samples from wild type and C4BPB -disrupted K562 cells (clone #5 in Fig. 2a ) were mixed in various ratios and subjected to RGEN-RFLP and T7E1 assays. Data points are represented as mean±s.e.m. of two independent experiments. Full size image Next, we designed and tested a new RGEN that targets a highly polymorphic locus, HLA-B , which encodes Human Leukocyte Antigen B (also known as MHC class I protein). HeLa cells were transfected with RGEN plasmids, and the genomic DNA was subjected to T7E1 and RGEN-RFLP analyses in parallel ( Fig. 4a ). T7E1 produced false-positive bands that resulted from sequence polymorphisms near the target site ( Fig. 4b ). As expected, however, the same RGEN used for gene disruption cleaved PCR products from wild-type cells completely but those from RGEN-transfected cells partially, indicating the presence of RGEN-induced indels at the target site. This result shows that RGEN-RFLP analysis has a clear advantage over the T7E1 assay, especially when it is not known whether target genes have polymorphisms or variations in cells of interest. 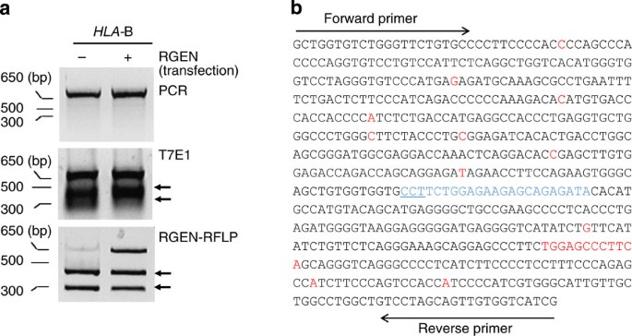Figure 4: Genotyping of RGEN-induced mutations at the highly polymorphicHLA-Blocus using RGEN-RFLP. (a) HeLa cells were transfected with aHLA-B-specific RGEN. RGEN-induced mutations were analysed using RGEN-RFLP and T7E1 assays in parallel. (b) The DNA sequence, which surrounds the RGEN target site, is that of a PCR amplicon from HeLa cells. Polymorphic positions are shown in red. The RGEN target site is shown in blue. The PAM sequence is underlined. Arrows indicate PCR primer sequences. Figure 4: Genotyping of RGEN-induced mutations at the highly polymorphic HLA-B locus using RGEN-RFLP. ( a ) HeLa cells were transfected with a HLA-B -specific RGEN. RGEN-induced mutations were analysed using RGEN-RFLP and T7E1 assays in parallel. ( b ) The DNA sequence, which surrounds the RGEN target site, is that of a PCR amplicon from HeLa cells. Polymorphic positions are shown in red. The RGEN target site is shown in blue. The PAM sequence is underlined. Arrows indicate PCR primer sequences. Full size image RGEN-mediated genotyping of ZFN and TALEN-induced mutations We then applied RGEN genotyping to the analysis of mutant mouse founders that had been established using a Pibf1 -specific TALEN [27] ( Supplementary Fig. 1 ). We designed and used two RGENs specific to the TALEN target site ( Fig. 5a ). One RGEN recognized the NGG PAM sequence and the other RGEN recognized the NAG PAM sequence. These two RGENs successfully detected various mutations, which ranged from 1–27-bp deletions. Unlike the T7E1 assay, RGEN genotyping enabled differential detection of heterozygous +/− founders (#4 and 5) from compound heterozygous −/− founders (#1, 3, 6, 8 and 11) ( Fig. 5a ). In addition, we used RGENs to detect mutations induced in human cells by a CCR5 -specific ZFN, representing yet another class of engineered nucleases ( Fig. 5b ). These results show that RGENs can detect mutations induced by nucleases other than RGENs themselves. In fact, we expect that RGENs can be designed to detect mutations induced by most, if not all, engineered nucleases. The only limitation in the design of an RGEN genotyping assay is the requirement for the GG or AG (CC or CT on the complementary strand) dinucleotide in the PAM sequence recognized by the Cas9 protein, which occurs once per 4 bp on average. Indels induced anywhere within the seed region of several bases in crRNA and the PAM nucleotides are expected to disrupt RGEN-catalyzed DNA cleavage. Indeed, we identified at least one RGEN site in most (98%) of the ZFN and TALEN sites we had reported previously [4] , [23] , [28] , [29] ( Supplementary Table 1 ). In contrast, only 36 sites (26%) have appropriate sites for RFLP analysis using conventional restriction enzymes. 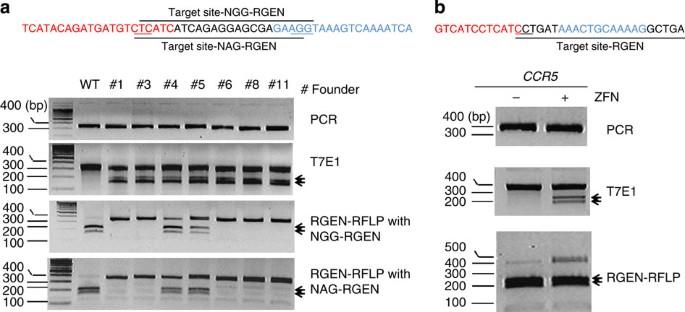Figure 5: RGEN-mediated genotyping of ZFN/TALEN-induced mutations. (a) Genotyping of mouse founders generated by aPIBF-targeting TALEN. The left and right half-sites of the PIBF TALEN are shown in red and blue, respectively. The PAM sequence recognized by Cas9 is underlined. (b) RGEN-mediated genotyping of ZFN-induced mutations. The left and right half-sites of the CCR5-ZFN are shown in red and blue, respectively. Black lines indicate RGEN target sites. Arrows indicate DNA bands cleaved by RGEN or T7E1. Figure 5: RGEN-mediated genotyping of ZFN/TALEN-induced mutations. ( a ) Genotyping of mouse founders generated by a PIBF -targeting TALEN. The left and right half-sites of the PIBF TALEN are shown in red and blue, respectively. The PAM sequence recognized by Cas9 is underlined. ( b ) RGEN-mediated genotyping of ZFN-induced mutations. The left and right half-sites of the CCR5-ZFN are shown in red and blue, respectively. Black lines indicate RGEN target sites. Arrows indicate DNA bands cleaved by RGEN or T7E1. Full size image RGEN-RFLP analysis of naturally occurring variations RGEN-RFLP analysis has applications beyond genotyping of engineered nuclease-induced mutations. We sought to use RGEN genotyping to detect recurrent mutations found in cancer and naturally occurring polymorphisms. We chose the human colorectal cancer cell line, HCT116, which carries a gain-of-function 3-bp deletion in the oncogenic CTNNB1 gene encoding beta-catenin [30] . PCR products amplified from HCT116 genomic DNA were cleaved partially by both wild-type-specific and mutant-specific RGENs, in line with the heterozygous genotype in HCT116 cells ( Fig. 6a ). In sharp contrast, PCR products amplified from DNA from HeLa cells harbouring only wild-type alleles were digested completely by the wild-type-specific RGEN and were not cleaved at all by the mutation-specific RGEN. 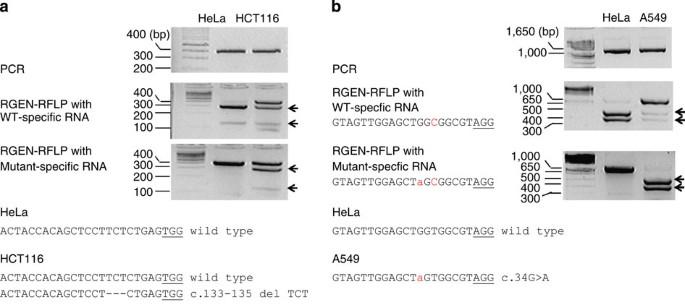Figure 6: Genotyping of oncogenic mutations via RGEN-RFLP analysis. (a) A recurrent mutation (c.133–135 deletion of TCT) in the humanCTNNB1gene in HCT116 cells was detected by RGENs. (b) Genotyping of theKRASsubstitution mutation (c.34G>A) in the A549 cancer cell line with RGENs that contain mismatched guide RNA. Mismatched nucleotides are shown in red. HeLa cells were used as a negative control. Arrows indicate DNA bands cleaved by RGENs. DNA sequences confirmed by Sanger sequencing are shown. Figure 6: Genotyping of oncogenic mutations via RGEN-RFLP analysis. ( a ) A recurrent mutation (c.133–135 deletion of TCT) in the human CTNNB1 gene in HCT116 cells was detected by RGENs. ( b ) Genotyping of the KRAS substitution mutation (c.34G>A) in the A549 cancer cell line with RGENs that contain mismatched guide RNA. Mismatched nucleotides are shown in red. HeLa cells were used as a negative control. Arrows indicate DNA bands cleaved by RGENs. DNA sequences confirmed by Sanger sequencing are shown. Full size image We also noted that HEK293 cells harbour the 32-bp deletion (del32) in the CCR5 gene, which encodes an essential co-receptor of HIV infection: Homozygous del32 CCR5 carriers are immune to HIV infection [31] . We designed one RGEN specific to the del32 allele and the other to the wild-type allele. As expected, the wild-type-specific RGEN cleaved the PCR products obtained from K562, SKBR3 or HeLa cells (used as wild-type controls) completely but those from HEK293 cells partially ( Supplementary Fig. 2a ), confirming the presence of the uncleavable del32 allele in HEK293 cells. Unexpectedly, however, the del32-specific RGEN cleaved the PCR products from wild-type cells as efficiently as those from HEK293 cells. Interestingly, this RGEN had an off-target site with a single-base mismatch immediately downstream of the on-target site ( Supplementary Fig. 2 ). These results suggest that RGENs can be used to detect naturally occurring indels but cannot distinguish sequences with single-nucleotide polymorphisms or point mutations due to their off-target effects. Genotyping of single-nucleotide variations via RGEN-RFLP To genotype oncogenic single-nucleotide variations [32] using RGENs, we attenuated RGEN activity by employing a single-base mismatched guide RNA instead of a perfectly matched RNA. RGENs that contained the perfectly matched guide RNA specific to the wild-type sequence or mutant sequence cleaved both sequences ( Supplementary Figs 3 and 4 ). In contrast, RGENs that contained a single-base mismatched guide RNA distinguished the two sequences, enabling genotyping of three recurrent oncogenic point mutations in the KRAS , PIK3CA and IDH1 genes in human cancer cell lines ( Fig. 6b and Supplementary Fig. 5a,b ). In addition, we were able to detect point mutations in the BRAF and NRAS genes using RGENs that recognize the NAG PAM sequence ( Supplementary Fig. 5c,d ). We believe that we can use RGEN-RFLP to genotype almost any, if not all, mutations or polymorphisms in the human and other genomes. Here we showed that RGEN-RFLP analysis can be used for genotyping both engineered nuclease-induced mutations and naturally occurring variations in cultured cells and animals. Unlike the T7E1 assay, RGEN-RFLP analysis is not limited by sequence polymorphisms near the nuclease target sites and distinguishes homozygous biallelic mutant clones from wild-type clones and heterozygous monoallelic mutant (+/−) clones from heterozygous biallelic mutant (−/−) clones. These features can make RGEN-RFLP a method of choice for detecting indels induced by RGENs and other nucleases. We observed, however, that RGENs often cannot distinguish off-target DNA sequences with a single-nucleotide mismatch. This off-target DNA cleavage by RGENs does not limit the utility of RGEN-RFLP for measuring the frequency of nuclease-induced mutations because error-prone non-homologous end-joining repair of DSBs rarely produces single-nucleotide substitutions. We employed attenuated guide RNAs that contain a single-base mismatch rather than perfectly matched guide RNAs to distinguish the wild-type sequences from the mutant sequences with substitutions. This result is consistent with our recent report that RGENs transfected into cultured human cells discriminate on-target sites from off-target sites that differ by two bases efficiently but not those that differ by a single base [33] . We also found that, at least partially due to off-target DNA cleavage, RGEN concentrations need to be optimized for each RFLP analysis ( Supplementary Table 2 ). Next-generation sequencing platforms are now widely used for genotyping in basic and biomedical research, including genotyping of mutations induced by engineered nucleases, and will soon be used broadly for diagnostics. RFLP analysis, however, may remain a method of choice in many settings, because it is a fast and inexpensive method with no requirement for special equipment. RGEN-RFLP analysis will broaden the utility of this convenient and robust method in a wide range of applications, enabling genotyping of both naturally occurring and nuclease-induced mutations. RGEN components crRNA and tracrRNA were prepared by in vitro transcription using MEGAshortcript T7 kit (Ambion) according to the manufacturer’s instruction. Transcribed RNAs were resolved on an 8% denaturing urea-PAGE gel. The gel slice containing RNA was cut out and transferred to elution buffer. RNA was recovered in nuclease-free water followed by phenol:chloroform extraction, chloroform extraction and ethanol precipitation. Purified RNA was quantified by spectrometry. Templates for crRNA were prepared by annealing an oligonucleotide whose sequence is shown as 5′-GAAATTAATACGACTCACTATAGGX 20 GTTTTAGAGCTATGCTGTTTTG-3′, in which X 20 is the target sequence, and its complementary oligonucleotide. The template for tracrRNA was synthesized by extension of forward and reverse oligonucleotides (5′-GAAATTAATACGACTCACTATAGGAACCATTC AAAACAGCATAGCAAGTTAAAATAAGGCTAGTCCG-3′ and 5′-AAAAAAAGCACCGACT CGGTGCCACTTTTTCAAGTTGATAACGGACTAGCCTTATTTTAACTTGCTATG-3′) using Phusion polymerase (New England Biolabs). Recombinant Cas9 protein Recombinant Cas9 protein was purchased from ToolGen, Inc. or purified from E. coli . The Cas9 DNA construct that encodes S. pyogenes Cas9 fused to the His 6 -tag at the C terminus was inserted in the pET-28a expression vector. The recombinant Cas9 protein was expressed in E. coli strain BL21(DE3) cultured in LB medium at 25 °C for 4 h after induction with 1 mM IPTG. Cells were harvested and resuspended in buffer containing 20 mM Tris (PH 8.0), 500 mM NaCl, 5 mM imidazole and 1 mM PMSF. Cells were frozen in liquid nitrogen, thawed at 4 °C and sonicated. After centrifugation, Cas9 protein in the lysate was bound to Ni-NTA agarose resin (Qiagen), washed with buffer containing 20 mM Tris (pH 8.0), 500 mM NaCl and 20 mM imidazole, and eluted with buffer containing 20 mM Tris (pH 8.0), 500 mM NaCl and 250 mM imidazole. Purified Cas9 protein was dialyzed against 20 mM HEPES (pH 7.5), 150 mM KCl, 1 mM DTT and 10% glycerol and analysed by SDS–PAGE. T7 endonuclease I assay The T7E1 assay was performed as described previously [23] . In brief, PCR products amplified using genomic DNA were denatured at 95 °C, reannealed at 16 °C and incubated with 5 units of T7 Endonuclease I (New England BioLabs) for 20 min at 37 °C. The reaction products were resolved using 2–2.5% agarose gel electrophoresis. The DNA sequences of PCR primers are shown in Supplementary Table 3. Full gel images are shown in Supplementary Figs 6–10 . RGEN-RFLP assay PCR products (100–150 ng) were incubated for 60 min at 37 °C with optimized concentrations (Supplmentary Table 2) of Cas9 protein, tracrRNA, crRNA in 10 μl NEB buffer 3 (1 × ). After the cleavage reaction, RNase A (4 μg) was added, and the reaction mixture was incubated for 30 min at 37 °C to remove RNA. Reactions were stopped with 6 × stop solution buffer containing 30% glycerol, 1.2% SDS and 100 mM EDTA. Products were resolved with 1–2.5% agarose gel electrophoresis and visualized with EtBr staining. Full gel images are shown in Supplementary Figs 6–10 . Plasmid cleavage assay Restriction enzyme-treated linearized plasmid (100 ng) was incubated for 60 min at 37 °C with Cas9 protein (0.1 μg), tracrRNA (60 ng) and crRNA (25 ng) in 10 μl NEB 3 buffer (1 × ). Reactions were stopped with 6 × stop solution containing 30% glycerol, 1.2% SDS and100 mM EDTA. Products were resolved with 1% agarose gel electrophoresis and visualized with EtBr staining. How to cite this article: Kim, J. M. et al. Genotyping with CRISPR-Cas-derived RNA-guided endonucleases. Nat. Commun. 5:3157 doi: 10.1038/ncomms4157 (2014).